Axonal and subcellular labelling using modified rabies viral vectors An important aspect of any neural circuit is the placement of its output synapses, at levels ranging from macroscopic to subcellular. The many new molecular tools for locating and manipulating synapses are limited by the viral vectors available for delivering them. Adeno-associated viruses are the best current means of labelling and manipulating axons and synapses, but they have never expressed more than one transgene highly enough to label fine axonal structure while also labelling or perturbing synapses. Their slow expression also makes them incompatible with retrograde and transsynaptic vectors, preventing powerful combinatorial experiments. Here we show that deletion-mutant rabies virus can be specifically targeted to cells local to an injection site, brightly labelling axons even when coexpressing two other transgenes. We demonstrate several novel capabilities: simultaneously labelling axons and presynaptic terminals, labelling both dendrites and postsynaptic densities, and simultaneously labelling a region’s inputs and outputs using co-injected vectors. Understanding the role of any circuit within the brain requires knowledge of where else in the nervous system it sends its output. As the major output pathways of almost all neurons are their axons, this is most straightforwardly achieved by imaging either the axons themselves or the synapses they form. Tools for ‘anterograde tracing’ or labelling the axons that emanate from some site of interest date back many decades [1] , and the ongoing development of molecular biological tools is allowing the mapping and manipulation of synapses in much greater detail [2] , [3] , [4] , [5] , [6] , [7] , [8] , [9] . However, the viral vectors that have so far been available for delivering these molecular tools to axons and synapses have significant limitations. The most prominent limitation of available ‘anterograde’ (that is, infecting cell bodies and delivering transgene products to axons) vectors is their inability to provide high-level expression of more than a single transgene [3] , [9] , [10] . Although multiple transgenes can of course be included in an adeno-associated virus (AAV), for example, to our knowledge there is no published example of any polycistronic viral vector that has simultaneously expressed any other transgene in combination with a cytoplasmic fluorophore expressed at levels high enough to allow clear visualization and reconstruction of axonal morphology. A recent such attempt illustrates the point: an AAV designed to express cytoplasmic mCherry along with a synaptobrevin-enhanced green fluorescent protein (EGFP) fusion resulted in cytoplasmic labelling only of the thickest axons, not the fine processes that are necessary, for example, to identify the cell bodies of origin of particular labelled synapses [11] . This inability of AAV to express multiple transgenes at high levels has prevented simple but powerful experiments such as simultaneously labelling synaptic locations and detailed axonal structure, or combining optogenetic confirmation of synaptic contacts with detailed reconstruction of axonal and dendritic architecture. The timescales of existing anterograde vectors are also problematic. The viral species typically used for labelling axons require weeks or even months for adequate expression [3] , [9] , [11] , whereas the few published alternatives with faster expression are so toxic that infected neurons sicken and die within 2–3 days [12] , [13] . It would therefore be difficult to combine any of these vectors with those that allow gene delivery by two other routes of equally great importance: retrograde (in which genes are delivered to projection neurons through their axons projecting to a remote injection site) and transsynaptic (in which a viral vector spreads to the target neurons from neurons in synaptic contact with them). This is because rabies viral (RV) vectors, which are the best current means of both transsynaptic and retrograde gene delivery [14] , [15] , [16] , [17] , [18] , [19] , [20] , [21] , [22] , [23] , have a working window that falls in the large gap between the very slow and very fast toxic ranges of the available anterograde vectors. The lack of compatible anterograde and retrograde or transsynaptic vectors has prevented powerful combinatorial experiments, such as optically stimulating incoming anterogradely targeted axons whereas imaging the resulting postsynaptic activity in retrogradely -targeted dendrites with cytoplasmic fluorophores allowing imaging and 3D reconstruction of these neurites. What is needed is an anterograde vector that, first, allows high-level expression of multiple transgenes and, second, does so on a timescale that matches that of retrograde and transsynaptic vectors. Here we show that deletion-mutant rabies virus (RV), which is ordinarily very efficient at retrogradely infecting distant neurons projecting to an injection site, can be transformed into a vector that specifically infects cells local to an injection site, simply by packaging it with the envelope protein of a different virus. This repackaging leaves intact its signature rapid, high and stereotyped transgene expression, so that axons can be brightly labelled with soluble fluorescent proteins, making them clearly individually resolvable. We also show that multiple transgenes can be incorporated into the RV genome with stereotyped expression levels that can be chosen based on the needs of the experiment. Single viral vectors can therefore be used to label multiple subcellular compartments, as in the example shown here of labelling both dendrites and postsynaptic densities of retrogradely targeted neurons, which has never before been demonstrated. We combine the above characteristics to demonstrate bright, multicolour fluorescent anterograde labelling of neurons’ axons and presynaptic terminals (which has itself never before been achieved) in addition to expression from the same viral vector of a third transgene, in this case used to label the neurons’ nuclei in a third colour. Because the timescale of expression from this anterograde version of RV matches those of the previously published retrograde and transsynaptic versions, the different vectors can be used in combination within the same subject for simultaneous gene delivery to different neuronal populations by different routes. This includes, as we show here, simultaneous tracing, in different colours, of both outputs and inputs of a region of interest by co-injecting anterograde and retrograde vectors. Packaging RV with VSVG abolishes retrograde infectivity We first investigated whether packaging RV vectors with the envelope glycoprotein of vesicular stomatitis virus (VSVG) would eliminate their usually marked propensity for retrogradely infecting remote neurons and instead target their infectivity to cells local to the injection site. This expectation seemed reasonable, because lentiviral vectors that are packaged with VSVG efficiently infect local neurons and glia but do not infect retrogradely when injected into the nervous system, whereas those that are instead packaged with the RV envelope glycoprotein (RVG) infect retrogradely with efficiency comparable to that of RV [14] , [24] (albeit with far lower expression levels). We generated a VSVG-enveloped rabies viral vector encoding EGFP [25] by growing the previously described RV-4GFP [26] in cells expressing a fusion protein comprising the extracellular and transmembrane domains of VSVG (Indiana strain) and the cytoplasmic domain of RVG [27] ; such substitution of the native RVG cytoplasmic tail increases the efficiency of incorporation into the envelopes of RV virions while preserving the tropism of the exogenous glycoprotein [15] , [28] , [29] . We equalized the titres of the VSVG-enveloped and RVG-enveloped preparations of RV-4GFP and injected equal volumes (20 nl) into the primary somatosensory cortex of different mice. 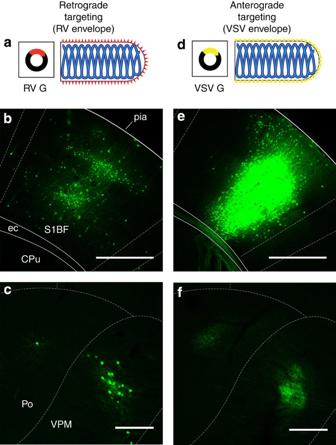Figure 1: Packaging deletion-mutant RV with the VSV envelope protein abolishes retrograde infectivity. (a) Schematic of packaging G-deleted RV with its own envelope protein for efficient infection of distant neurons projecting to an injection site, as described in Wickershamet al.26(b) Injection site in mouse barrel cortex of RV-4GFP packaged with RV G. Many cortical neurons with cell bodies distant from the injection site are labelled. (c) Numerous retrogradely infected cells are also present in the somatosensory thalamus (VPM and Po nuclei) of the same mouse. (d) Schematic packaging of G-deleted RV with the VSV envelope protein for local instead of retrograde infection. (e) Injection site in mouse barrel cortex of RV-4GFP packaged with VSV G, with injection volume and viral titre equal to those of the injection depicted in panelsbandc. Infected neurons are restricted to a tight cluster at the injection site, with bright GFP labelling of their axons. (f) The somatosensory thalamus of the same animal contains dense arbourizations of cortical axons in VPM and Po brightly labelled with GFP, but no retrogradely labelled cell bodies. Overlays indicating approximate structural boundaries are adapted from Franklinet al.60S1BF,primary somatosensory cortex, barrel field; ec, external capsule; CPu, caudate putamen; Po, posterior thalamic nuclear group; VPM, ventral posteromedial thalamic nucleus. Scale bars,bande500 μm,candf200 μm. Figure 1 depicts the results. As described previously [14] , the RV enveloped with its native glycoprotein (schematically depicted in Fig. 1a ) retrogradely infected neurons spread widely throughout the brain. At the injection site in the cortex ( Fig. 1b ), labelled neurons were found diffusely, with distribution extending laterally from the injection site in layer 5 (the location of which is indicated by the presence of fluorescent glia) and a striking blade of labelled neurons in layer 2/3, consistent with the known projection from this layer to layer 5 (ref. 30 ). In thalamus, retrogradely infected relay neurons were found in the somatosensory nuclei ( Fig. 1c ), with most found in the ventral posteromedial nucleus (VPM, primary somatosensory nucleus) and smaller numbers in the posterior nucleus (Po, secondary somatosensory nucleus). Figure 1: Packaging deletion-mutant RV with the VSV envelope protein abolishes retrograde infectivity. ( a ) Schematic of packaging G-deleted RV with its own envelope protein for efficient infection of distant neurons projecting to an injection site, as described in Wickersham et al . [26] ( b ) Injection site in mouse barrel cortex of RV-4GFP packaged with RV G. Many cortical neurons with cell bodies distant from the injection site are labelled. ( c ) Numerous retrogradely infected cells are also present in the somatosensory thalamus (VPM and Po nuclei) of the same mouse. ( d ) Schematic packaging of G-deleted RV with the VSV envelope protein for local instead of retrograde infection. ( e ) Injection site in mouse barrel cortex of RV-4GFP packaged with VSV G, with injection volume and viral titre equal to those of the injection depicted in panels b and c . Infected neurons are restricted to a tight cluster at the injection site, with bright GFP labelling of their axons. ( f ) The somatosensory thalamus of the same animal contains dense arbourizations of cortical axons in VPM and Po brightly labelled with GFP, but no retrogradely labelled cell bodies. Overlays indicating approximate structural boundaries are adapted from Franklin et al . [60] S1BF,primary somatosensory cortex, barrel field; ec, external capsule; CPu, caudate putamen; Po, posterior thalamic nuclear group; VPM, ventral posteromedial thalamic nucleus. Scale bars, b and e 500 μm, c and f 200 μm. Full size image In sharp contrast, infection by the RV enveloped with the VSV glycoprotein ( Fig. 1d–f ) was restricted to a tight cluster of cells at the injection site ( Fig. 1e ). As seen in Fig. 1b,e , injection of the VSVG-enveloped vector resulted in a far denser labelling of neurons at the injection site than did injection of the RVG-enveloped version. This is presumably because the neurons infected by the VSVG-enveloped vector were almost entirely restricted to the injection site, whereas a large proportion of the neurons infected by the RVG-enveloped vector (which was matched in titre and injection volume) were remote projection neurons infected through their axon terminals at the injection site. There were no retrogradely infected cells in the thalamus ( Fig. 1f ), only dense arbours of GFP-filled axons in both VPM and Po, matching the locations of retrogradely labelled relay neurons in the previous case. Supplementary Fig. S1 shows close-ups of these anterogradely labelled axons, with very different morphologies of axons and terminals seen in the projections to the two different thalamic nuclei. Neurons retrogradely labelled by the VSVG-enveloped RV were very rarely seen (one found in superficial layer 2 of the ipsilateral sensorimotor cortex 1.5 mm anterior to the injection site is shown in Supplementary Fig. S2 ). However, this residual retrograde infectivity (which is also seen with AAV [31] , [32] , [33] ) was not a major feature, with never more than two labelled neurons found in contralateral cortex, and none found in the thalamus, in any animal. Expression level depends on location in the RV genome Next, we quantified the expression levels of transgenes located at different loci within the RV genome, in order to better inform decisions of vector design for experiments requiring expression of multiple transgenes. We expected the expression levels of transgenes to depend on their locations in the viral genome, because the expression levels of the five endogenous rabies viral genes have been shown to decrease monotonically with increasing distance from the start (3′ end) of the negative-strand RNA genome [34] . All previously published G-deleted rabies viral vectors contained one or two transgenes located in the position of the deleted glycoprotein gene between the viral matrix and polymerase genes [14] , [26] , [35] , [36] , [37] . We have now inserted an additional transgene locus at the start of the viral genome, immediately following the leader sequence and before the viral nucleoprotein gene. We expected that this would result in the highest possible transgene expression in addition to allowing the inclusion of a third transgene in a single vector. We constructed an array of rabies viral vectors to compare the expression levels of transgenes located in these three positions. These vectors constituted a complete set, with all possible combinations of either zero or one transgene at the genome start, and zero, one or two transgenes in the place of G, with EGFP appearing as one of the transgenes in each possible position and with other transgenes included as placeholders as required ( Fig. 2a ). We infected wells of HEK-293T cells with equal amounts of these vectors and quantified the intensity of the resulting fluorescence by flow cytometry (sample fluorescence histograms are shown in Supplementary Fig. S3 ). As predicted, the expression from the various vectors was at stereotyped and distinct levels, with intensity decreasing with distance from the genome start. EGFP was expressed from the leader-proximal locus at a much higher level than from the previously used loci in the position of the deleted G: fluorescence resulting from the highest-expressing vector (vector iv in Fig. 2a ) was 2.4-fold higher than that resulting from the single-gene version (vector i, previously described in Wickersham et al . [26] ), and 2.7-fold and 2.9-fold higher than the two versions with two transgenes only in the G locus (vectors ii and iii), as in previously published vectors [37] . Furthermore, addition of the new leader-proximal locus decreased the expression level of genes (either one or two) in the original G locus, by 30% in the case of a single gene (vector vii versus vector i) and 29 and 22% in the two gene cases (vector viii versus vector ii, and vector ix versus vector iii). All these differences were highly significant (pair wise two-tailed t -tests, P <0.0001). Supplementary Table S1 contains the brightness means, standard deviations, numbers of fluorescent cells, standard errors of the means, t values and degrees of freedom for all of the above comparisons. 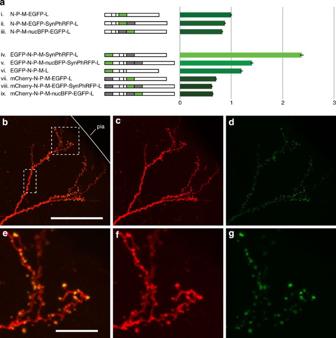Figure 2: Expression of multiple transgenes from single vectors allows simultaneous labelling of neurites and synapses. (a) Transgene location within the viral genome determines expression level, as determined by flow cytometric analysis of EGFP brightness. Two transgenes inserted in the G locus have only slightly lower expression than a single one. Addition of a transgene in the promoter-proximal locus prior to the first viral gene, with a second transgene in the original G locus, results in expression 2.4-fold higher than that of a single gene in the G locus. Error bars denote standard error of the mean (n=1550–2873; see Methods). (b,c) Two-colour brightly fluorescent labelling of the apical dendrites and postsynaptic densities of a layer 5 cortical pyramidal cell. Cytoplasmic mOrange2 is expressed at a high level from the promoter-proximal locus; PSD-95-EGFP fusion is expressed at a lower level from the G locus. Solid line indicates approximate location of pia; dashed square indicates region enlarged in panels (d,e); dashed rectangle indicates region enlarged inSupplementary Fig. S4. (d,e) Higher-resolution image of region enclosed by dashed square in panelb. EGFP puncta are located on dendritic spines. Scale bars,b–d50 μm,e–g10 μm. Figure 2: Expression of multiple transgenes from single vectors allows simultaneous labelling of neurites and synapses. ( a ) Transgene location within the viral genome determines expression level, as determined by flow cytometric analysis of EGFP brightness. Two transgenes inserted in the G locus have only slightly lower expression than a single one. Addition of a transgene in the promoter-proximal locus prior to the first viral gene, with a second transgene in the original G locus, results in expression 2.4-fold higher than that of a single gene in the G locus. Error bars denote standard error of the mean ( n =1550–2873; see Methods). ( b , c ) Two-colour brightly fluorescent labelling of the apical dendrites and postsynaptic densities of a layer 5 cortical pyramidal cell. Cytoplasmic mOrange2 is expressed at a high level from the promoter-proximal locus; PSD-95-EGFP fusion is expressed at a lower level from the G locus. Solid line indicates approximate location of pia; dashed square indicates region enlarged in panels ( d , e ); dashed rectangle indicates region enlarged in Supplementary Fig. S4 . ( d , e ) Higher-resolution image of region enclosed by dashed square in panel b . EGFP puncta are located on dendritic spines. Scale bars, b – d 50 μm, e – g 10 μm. Full size image Labelling both dendrites and postsynaptic densities We took advantage of this ability to express multiple transgenes at defined and stereotyped levels to engineer vectors to simultaneously label different subcellular compartments of neurons. As an example, we constructed a genome with the sequence encoding mOrange2 (ref. 38 ) in the leader-proximal locus and a gene encoding a fusion protein of PSD-95 (ref. 39 ) and EGFP in the G locus and packaged this genome with the native RVG for retrograde delivery. Figure 2b–g depicts the apical dendrites of a layer 5 barrel cortical pyramidal cell retrogradely infected from an injection in the somatosensory thalamus. The vector brightly labels the detailed structure of dendrites with the cytoplasmically soluble mOrange2, whereas the PSD-95-EGFP fusion results in punctate labelling along dendrites and prominent on dendritic spines. Labelling of axons and synaptic terminals as well as nuclei We combined these two abilities of RV – anterograde targeting, and expression of multiple transgenes at defined levels – to create an anterograde tracing tool for simultaneous multicolour fluorescent labelling of three separate subcellular compartments: first, axonal processes, to illuminate projection pathways and allow reconstruction of individual axons, second presynaptic terminals, to indicate the exact locations of synapses, and, third, the neurons’ nuclei, for easily counting infected neurons to provide a ‘normalization factor’ allowing quantitative comparison of the results of different injections [9] . We constructed a genome with the EGFP gene in the leader-proximal locus and two other transgenes in the G locus, the first encoding a nuclearly localized version of the bright blue fluorophore mTagBFP [40] and the second encoding a fusion protein of synaptophysin [41] and the bright red fluorophore TagRFP-T [38] (genome v in Fig. 2a ). We packaged this genome with the VSV envelope protein for local infectivity and made 5-nl injections into mouse somatosensory cortex. 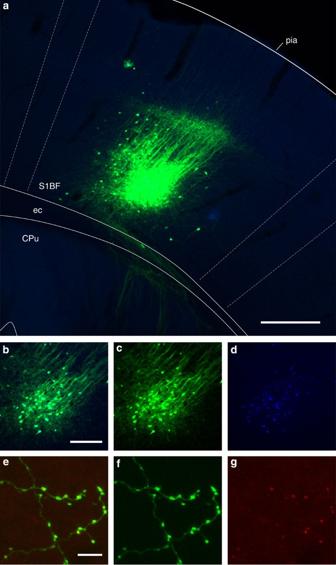Figure 3: Simultaneous multicolour brightly fluorescent labelling of three subcellular compartments. (a) Injection site in mouse somatosensory cortex of anterograde (locally infecting) rabies virus encoding cytoplasmic EGFP, nuclearly localized mTagBFP and synaptophysin-TagRFP-T fusion protein. A tight cluster of cells primarily in layer 6 resulted from this 5 nl injection, with little labelling in more superficial layers. Descending and locally arbourizing axons are brightly labelled. Overlay indicating approximate structural boundaries is adapted from Franklinet al.60(b–d) Higher-power image of the layer 6 cells, with separate green and blue channels showing cytoplasmic EGFP and nuclear mTagBFP. (e-g) High-power image of thalamocortical axonal processes (green) and synaptic terminals (red) in the primary somatosensory thalamus (ventral posteriomedial nucleus). S1BF, primary somatosensory cortex, barrel field; ec, external capsule; CPu, caudate putamen. Scale bars,a250 um,b–d100 μm,e–g5 μm. Figure 3 depicts the results. Figure 3: Simultaneous multicolour brightly fluorescent labelling of three subcellular compartments. ( a ) Injection site in mouse somatosensory cortex of anterograde (locally infecting) rabies virus encoding cytoplasmic EGFP, nuclearly localized mTagBFP and synaptophysin-TagRFP-T fusion protein. A tight cluster of cells primarily in layer 6 resulted from this 5 nl injection, with little labelling in more superficial layers. Descending and locally arbourizing axons are brightly labelled. Overlay indicating approximate structural boundaries is adapted from Franklin et al . [60] ( b – d ) Higher-power image of the layer 6 cells, with separate green and blue channels showing cytoplasmic EGFP and nuclear mTagBFP. ( e - g ) High-power image of thalamocortical axonal processes (green) and synaptic terminals (red) in the primary somatosensory thalamus (ventral posteriomedial nucleus). S1BF, primary somatosensory cortex, barrel field; ec, external capsule; CPu, caudate putamen. Scale bars, a 250 um, b – d 100 μm, e – g 5 μm. Full size image At the injection site (panels a–d), a tightly focused cluster of neurons, mostly layer 6 pyramidal cells with apical dendrites ascending to and ramifying in layer 4, is brightly labelled with EGFP. Even at low magnification (panel a), axons can be clearly seen traversing en masse through the white matter and descending in distinct groups through the striatum. At higher magnification ( × 25, panels b–d), individual neurons are clearly resolvable, particularly in the blue channel in which nuclei are distinctly labelled. In this field, 71 BFP-labelled nuclei are resolvable, with all but 4 (94.4%) unambiguously colocalized with EGFP-labelled somata. High-power ( × 100, panels e–g) imaging of the somatosensory thalamus (VPM) reveals that the EGFP-labelled fine processes of axonal arbours are easily resolvable, with punctate red fluorescence from the synaptophysin-TagRFP-T fusion protein colocalized with varicosities on the axons. Two-colour fluorescent labelling of inputs and outputs We then examined whether the novel anterograde RV vector could be used in combination with the previously published retrograde version, and, specifically, whether it was possible to jointly trace both the inputs and the outputs of a brain region by injecting a mixture of two viral vectors. This represents a powerful combinatorial assay much more informative than separately labelling inputs and outputs in different animals, because it would allow determination of the precise spatial register of outgoing axons with the dendrites of neurons projecting to the injection site, in any of the many cases of reciprocal connections between nuclei within the brain. We injected into mouse somatosensory thalamus (VPM) an equal mixture of two rabies viral vectors: one anterograde (VSVG enveloped) and encoding mOrange2 (ref. 38 ), the other retrograde (RVG enveloped) and encoding mCherry [42] . The results are shown in Fig. 4 . At the injection site in the thalamus, many relay neurons as well as glia were brilliantly labelled with mOrange2 ( Fig. 4a,b ). These neurons’ axons heavily innervated primary somatosensory cortex ( Fig. 4d,e ), running along the subcortical white matter before ascending through layers 6 and 5 and ramifying densely in layer 4 ( Fig. 4d,e ). By contrast, the retrograde virus labelled few cell bodies, but many processes, at the thalamic injection site ( Fig. 4a,c ). While some cells were co-infected by the two viruses (although some of the apparent mCherry fluorescence in the thalamus may be due to spectral overlap from the intense mOrange2 expression in cell bodies and processes there), most were not. This is most obvious in the cortex ( Fig. 4d–f ) where the vast majority of mOrange2-labelled thalamocortical axons did not express mCherry. However, many layer 6 pyramidal cells were retrogradely labelled with mCherry, in precise topographic register with the mOrange2-labelled thalamocortical projection. These cells’ apical dendrites ascended to layer 4 and terminated there, in the region of densest thalamocortical axonal ramification. 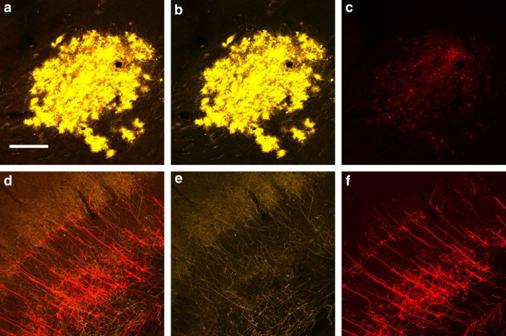Figure 4: Joint retrograde and anterograde tracing of inputs and outputs of a brain region. (a–c) Injection site in mouse somatosensory thalamus of an equal mixture of two deletion-mutant rabies viral vectors: VSVG-enveloped vector encoding mOrange2 (yellow), and an RVG-enveloped vector encoding mCherry (red). The VSVG-enveloped vector prolifically infects thalamic neurons at the injection site, whereas the RVG-enveloped one infects far fewer cells locally. (d–f) In the somatosensory cortex of the same mouse, mOrange2-filled thalamocortical axons ascend to layer 4 and densely ramify among the apical dendrites of mCherry-filled layer 6 corticothalamic cells retrogradely infected by the co-injected retrograde virus. Scale bar, 200 μm, applies to all panels. Figure 4: Joint retrograde and anterograde tracing of inputs and outputs of a brain region. ( a – c ) Injection site in mouse somatosensory thalamus of an equal mixture of two deletion-mutant rabies viral vectors: VSVG-enveloped vector encoding mOrange2 (yellow), and an RVG-enveloped vector encoding mCherry (red). The VSVG-enveloped vector prolifically infects thalamic neurons at the injection site, whereas the RVG-enveloped one infects far fewer cells locally. ( d – f ) In the somatosensory cortex of the same mouse, mOrange2-filled thalamocortical axons ascend to layer 4 and densely ramify among the apical dendrites of mCherry-filled layer 6 corticothalamic cells retrogradely infected by the co-injected retrograde virus. Scale bar, 200 μm, applies to all panels. Full size image We have shown here that packaging G-deleted RV with the VSV envelope protein, instead of the native RV one, almost completely removes its otherwise notable ability to infect retrogradely and causes it instead to efficiently infect local neurons. Because the tropism of VSVG-enveloped RV is determined by the VSV envelope protein itself, it can be expected to be pantropic and, furthermore, to work in a wide variety of taxa, including primates [43] , birds [44] and insects [45] . Despite its redirected tropism, the VSVG-enveloped version of RV retains the high and rapid transgene expression characteristic of the original, because the vectors are identical apart from their means of reaching the cytoplasm. For the same reason, we expect that the time courses of transgene expression levels and host cell toxicity are also similar. Here we have illustrated RV vectors’ ability to co-express multiple transgenes at stereotyped but differing levels ( Fig. 2a ) by constructing a vector to co-express cytoplasmic mOrange2 and a PSD-95-EGFP fusion protein ( Fig. 2b–g ). This constitutes the first published case of simultaneously labelling both dendrites and the postsynaptic sites on them by means of any retrograde vector. We expect vectors of this kind to be very useful tools in their own right for a number of important applications, such as rapid quantification of synaptic scaling along the dendritic branches of single neurons, a critical determinant of the integrative properties of dendritic arbours [46] . It is entirely possible that the expression levels of synaptic fusion proteins are excessive when these transgenes are located in the original G locus, as in the example vectors we have presented here. Overexpression of PSD-95, in particular, can be perturbative [47] , although, to the extent to which we have quantified synaptic density here (counting the PSD-95-EGFP-labelled puncta in Supplementary Fig. S4 ), it appears in line with the other published data [48] , [49] , [50] . Similarly, the 2.4-fold increase of EGFP expression resulting from placement of the new locus in the promoter-proximal position (where the EGFP gene also has been positioned in VSV vectors [12] and, unsuccessfully, in replication-competent RV [51] ) may be overkill, because EGFP expressed from the G locus is already sufficient for labelling fine axonal processes [14] , [16] , and even EGFP can be toxic at high levels [52] . It may therefore be desirable to design future vectors for lower transgene expression levels. We have shown here that multiple transgenes placed in the G locus are expressed at levels only slightly lower than those of single-transgene versions. Expression could be lowered further by straightforward means. Just as, as we have shown here, expression can be increased by moving transgenes closer to the start of the RV genome, it could as easily be decreased simply by moving them farther away, with loci added at the end of the genome (after the viral polymerase gene) expected to result in expression considerably lower than from any of the loci used here or in any previous deletion-mutant RV vectors. Furthermore, it should be possible to engineer arbitrarily low – but still stereotyped expression levels by the insertion of multiple such loci (even empty ones consisting only of transcriptional start and stop signals, included only as spacers to decrease expression of downstream transgenes) at the 5′ end of the viral genome. Our use of a VSVG-enveloped RV vector for multicolour labelling of axons, synaptic terminals and nuclei of neurons at an injection site ( Fig. 3 ) is innovative in several ways. First, simultaneously labelling axonal fine structure and synaptic terminals using a single viral vector has not previously been demonstrated, despite attempts to do so [11] . We have not only achieved this but also included a third transgene, in this case for labelling nuclei as well. Second, to our knowledge, this is the first published demonstration that three transgenes can be expressed from a single RV vector. This allows great flexibility in experimental design. Here we have used this option of a third transgene simply for expressing a third, nuclearly localized fluorophore, which would be useful in cases in which rapid counting of labelled neurons is needed for comparison of different injections [9] . Alternatively, this third transgene locus could be used instead for expression of channelrhodopsin, a calcium indicator, or indeed any other transgene [20] , [21] , [37] . Although there may be as-yet-unclear practical limits on the lengths of rabies viral vector genomes, there appears to be no hard constraint. The largest one that we have constructed for this work (genome v in Fig. 2 and used for the injections shown in Fig. 3 ) contains transgenes totalling 3,228 bases (720, 813 and 1,695 bases for EGFP, nuclearly localized BFP, and synaptophysin-TagRFP-T, respectively) for a total length of 13,353 bases (versus 11,928 bases for the wild-type SAD B19 genome [53] ). However, RV vectors containing two transgenes totalling up to 6.5 kb have previously been constructed, even without deleting the glycoprotein gene as we have done with all of the vectors presented here [54] . Simultaneously labelling the axons proceeding from a region of interest while also labelling the remote neurons sending projections to it, as we have demonstrated here, has not previously been achieved with any combination of viral vectors. In theory, this could be possible using other viral species, such as an AAV for anterogradely labelling axons co-injected with an HSV vector for retrogradely labelling projection neurons [55] . Assuming expression levels from such retrograde infection with an HSV are high enough for clear labelling of fine dendritic processes, this would presumably have the advantage of lower toxicity, which would be very useful for long-term studies. However, using RV vectors has two major advantages. The first and most obvious is the ability to express multiple transgenes at high levels, as discussed above. The second, however, is the notable lack of co-infection seen when the two RV variants are co-injected (Fig. 4 ), with the VSVG-enveloped anterograde virus evidently outcompeting the RVG-enveloped retrograde virus for infection of cells local to the injection site. This seems to be an example of the ‘superinfection interference’ that is a prominent feature of (even intracellularly) replication-competent viruses and which is seen also with intact RV [51] . Often a nuisance (hindering double-labelling studies, for example), in this case it allows not just simultaneous tracing of both outputs and inputs of a region of interest, but also largely non-overlapping expression of different transgenes in the two populations, so that the thalamocortical axons (panel e) do not express the transgene labelling the dendrites of the corticothalamic cells (panel f) and vice versa. This therefore would allow many other powerful combinatorial assays of reciprocal connections, such as including synaptic markers similar to those used in Figs. 2 and 3 for identification of putative synaptic contacts between the labelled axons and dendrites, or all-optical interrogation of the thalamo-cortico-thalamic circuit by expressing opsins in thalamocortical axons and expressing activity indicators in corticothalamic dendrites. We have here demonstrated that, in addition to the previously described retrograde [14] , transsynaptic [15] and genetic [15] , [56] delivery routes, rabies viral vectors can also be engineered to target neurons by a fourth route: anterograde delivery of transgene products to axons (see Fig. 5 ). With the additional ability to express multiple transgenes in each of the vectors used to target distinct neuronal populations by any of these four routes, this opens the door to focal identification and interrogation of synapses throughout the brain. One possible paradigm would be to express GRASP components [4] , [6] , [8] – the use of which has so far been restricted to application-specific transgenic and knock-in animals – in a wide range of putatively presynaptic and postsynaptic populations, for example, by anterograde and retrograde targeting, respectively. Alternatively, one could anterogradely label several separate inputs to a region by injecting different vectors in the nuclei that give rise to them, causing expression of different opsins in these various groups of axons, allowing their independent optical activation and determination of their effect on postsynaptic neuronal populations targeted retrogradely or transsynaptically for expression of calcium or voltage indicators, with co-expressed cytoplasmic fluorophores allowing three-dimensional reconstruction of all the neurites involved. Because as demonstrated here, these vectors can incorporate even three transgenes, the above paradigms could furthermore be combined to allow structural and functional interrogation of exactly the same circuits. These combinatorial possibilities are limited only by the spectral separation of fluorophores, activators and indicators, a barrier that is rapidly eroding with the ongoing development and refinement of these molecular tools. 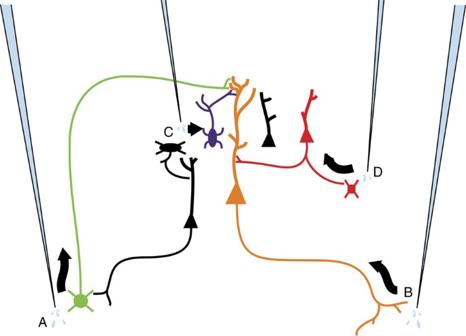Figure 5: Strategies now available for targeting multiple neuronal populations with different RV vector classes. (a) Anterograde targeting with VSVG-enveloped RV, introduced in this paper. (b) Retrograde targeting with RVG-enveloped RV14. (c) Genetic targeting with EnvA-enveloped RV15. Packaging RV with an avian retroviral envelope protein renders it unable to infect mammalian cells in the absence of engineered expression of an exogenous receptor. (d) Monosynaptic targeting with RV15. When complemented by engineered expression of RVGin trans, G-deleted RV spreads to neurons directly presynaptic to the G-expressing cells. Figure 5: Strategies now available for targeting multiple neuronal populations with different RV vector classes. ( a ) Anterograde targeting with VSVG-enveloped RV, introduced in this paper. ( b ) Retrograde targeting with RVG-enveloped RV [14] . ( c ) Genetic targeting with EnvA-enveloped RV [15] . Packaging RV with an avian retroviral envelope protein renders it unable to infect mammalian cells in the absence of engineered expression of an exogenous receptor. ( d ) Monosynaptic targeting with RV [15] . When complemented by engineered expression of RVG in trans , G-deleted RV spreads to neurons directly presynaptic to the G-expressing cells. Full size image Cloning All viral genome plasmids were derived from cSPBN [57] (itself derived from the SAD B19 genome plasmid pSAD L16 (ref. 58 )), with the glycoprotein gene deleted in all cases. For some vectors (such as the bottom six genomes depicted in Fig. 2a ), an additional open reading frame was inserted between the viral leader sequence and the nucleoprotein gene. All vectors had either one or two transgenes cloned into the G locus, with the exception of RV-1E (sixth genome from top in Fig. 2a ), for which the G locus (including start and stop sequences) was deleted entirely. The nuclearly localized blue fluorescent protein gene was constructed by cloning the mTagBFP [40] gene in frame with the nuclear localization signal (SV40 large T antigen triple tandem repeat) from pEYFP-Nuc (Clontech, Mountain View, CA). The fusion protein of PSD-95 with EGFP [25] was constructed by cloning the rat PSD-95 gene [59] in frame with that of EGFP. The fusion protein of synaptophysin with TagRFP-T [38] was constructed by de novo synthesis of the mouse synaptophysin gene [41] (GenBank accession number X95818 ) in frame with that of TagRFP-T. Gene synthesis and many cloning steps were performed by Epoch Life Science (Missouri City, TX). Vector production Vector production subsequent to cloning was performed by co-transfection of viral genome and helper plasmids followed by amplification by passaging in complementing cells [26] but using the BSR-VSV-RV-G cell line [27] instead of the BHK-B19G2 line [26] for the anterograde vectors. For vectors with a transgene preceding the nucleoprotein gene (for example, the last six genomes depicted in Fig. 2a ), supernatants were collected for one additional day (that is, at 48, 72 and 96 h following infection). Vectors were concentrated and purified by ultracentrifugation (2 h at 51,000 g , Thermo Surespin 630 rotor) of supernatants, with virus extracted from the interface of 20 and 60% sucrose solutions (w/v in Dulbecco’s phosphate-buffered saline DPBS), diluted in DPBS and pelleted by a second round of ultracentrifugation to remove sucrose, resuspended in DPBS and stored in 5–20 ul aliquots at −80°C. Titre determination and flow cytometric analysis HEK-293T cells (ATCC # CRL-11268) in 24-well plates were infected with serial dilutions [26] with medium changed 20 h after infection and cells resuspended in 1% paraformaldehyde after 3 days. Suspensions were analysed on a BD LSR II flow cytometer (BD Biosciences, San Jose, CA), with fluorescent cells’ brightness means and variances calculated using BD FACSDiva software. For t -tests, sample sizes for the nine groups were determined by the fraction of the total number of analysed cells (30,000 in each group) that was positive for EGFP fluorescence; these sample sizes were: i (4GFP) 2,553, ii (4E5S) 1,893, iii (4nB5E) 2,209, iv (1E5S) 1,732, v (1E5nB6SR) 1,660, vi (1E) 1,561, vii (1mC5E) 1,550, viii (1mC5E6S) 2,820, ix (1mC5nB6E) 2,873. Stereotaxic injections All work with animals was approved by the MIT Committee for Animal Care. Vectors were injected into either the primary somatosensory cortex (−0.58 AP, +3.0 LM, −1.75 DV, mm, relative to the bregma) or ventral posteromedial nucleus (−1.82 AP, +1.75 LM, −3.5 DV) of anesthetized adult male C57BL/6J mice (Jackson Laboratory, Bar Harbour, ME) using a stereotaxic instrument (Stoelting Co., Wood Dale, IL) and an injection mechanism consisting of a hydraulic manipulator (MO-10; Narishige Group, Tokyo, Japan) with headstage coupled via a custom adaptor to a wire plunger advanced through the pulled glass capillaries (Wiretrol II, Drummond) back-filled with mineral oil and front-filled with vector stock solution. For the matched injections of RVG- and VSVG-enveloped vectors ( Fig. 1 ), titres of both stocks were normalized to 2.0E10 IU ml −1 , with 20 nl (4E5 IU) of either stock injected per animal ( n =5 in each case). For retrograde bicolour labelling of dendrites and postsynaptic densities ( Fig. 2 ), 200 nl of virus (5.4E8 IU ml −1 , 1.1E5 IU total) was injected into VPM ( n =1). For anterograde tricolour labelling of axons, nuclei and presynaptic terminals ( Fig. 3 ), 5 nl of virus (8.6E9 IU ml −1 , 4.3E4 IU total) was injected into cortex ( n =2). For the joint injections of anterograde and retrograde vectors ( Fig. 4 ), a mixture containing 8.0E8 IU ml −1 of each was prepared and 50 nl (4.0E4 IU of each vector) injected per animal ( n =2). Histology and imaging Six to seven days following vector injection, mice were perfused transcardially with 4% paraformaldehyde in phosphate-buffered saline. Brains were postfixed in 4% paraformaldehyde overnight at 4 o C and cut into 50 μm coronal sections using a vibrating microtome (VF-700; Precisionary Instruments, San Jose, CA). Sections were mounted on Superfrost Plus slides (Fisher Scientific, Pittsburg, PA) with Prolong Gold Antifade mounting medium (Life Technologies, Grand Island, NY) and imaged on Olympus (Tokyo, Japan) FV1000 and Zeiss (Jena, Germany) LSM 710 confocal microscopes. Accession codes: Complete sequences of the genome plasmids for all vectors described in this manuscript have been deposited in the Genbank nucleotide database under accession codes KF450798 to KF450808 . How to cite this article: Wickersham, I. R. et al . Axonal and subcellular labelling using modified rabies viral vectors. Nat. Commun. 4:2332 doi: 10.1038/ncomms3332 (2013).